The Menin–Bach2 axis is critical for regulating CD4 T-cell senescence and cytokine homeostasis Although CD4 T-cell senescence plays an important role in immunosenescence, the mechanism behind this process remains unclear. Here we show that T cell-specific Menin deficiency results in the premature senescence of CD4 T cells, which is accompanied by the senescence-associated secretory phenotype after antigenic stimulation and dysregulated cytokine production. Menin is required for the expansion and survival of antigen-stimulated CD4 T cells in vivo and acts by targeting Bach2 , which is known to regulate immune homeostasis and cytokine production. Menin binds to the Bach2 locus and controls its expression through maintenance of histone acetylation. Menin binding at the Bach2 locus and the Bach2 expression are decreased in the senescent CD4 T cells. These findings reveal a critical role of the Menin-Bach2 pathway in regulating CD4 T-cell senescence and cytokine homeostasis, thus indicating the involvement of this pathway in the inhibition of immunosenescence. Age-induced alterations of innate and adaptive immunity are generally viewed as detrimental and designated as ‘immunosenescense’ [1] . Immunosenescence particularly affects the T-cell compartment and is involved in the age-related decline of immune functions, which increase the susceptibility of elderly individuals to infectious diseases and certain cancers [2] , [3] . Further, immunosenescence induces a pro-inflammatory state and increases the susceptibility to autoimmune diseases such as rheumatoid arthritis [4] , [5] . Evidence indicates that a prominent effect of ageing on immunity is reduced humoral responses, and that ageing is accompanied by alterations of the CD4 T-cell immunity [6] , [7] . Therefore, understanding immunosenescence requires knowledge of the age-associated alterations of CD4 T-cell functions and induction of cellular senescence. CD4 T-cell senescence represents a subset of cellular senescence, which is characterized by irreversible proliferation arrest caused by oxidative stress, reactive oxygen species, oncogene activity or the inactivation of tumour suppressor genes [8] , [9] . These factors contribute to tumour suppression, wound healing and ageing [9] . Senescent cells can significantly harm the tissue microenvironment through the acquisition of a senescence-associated secretory phenotype (SASP), which is characterized by a striking increase in the secretion of pro-inflammatory cytokines, chemokines, matrix remodelling factors and pro-angiogenic factors [10] , [11] . These factors deleteriously alter tissue homeostasis, leading to chronic inflammation and cancer [8] , [10] , [12] , [13] . Therefore, cellular senescence may contribute to a component of age-associated inflammatory responses called ‘inflammaging’ [14] . Certain germinal mutations of MEN1 , which encodes MENIN, cause multiple endocrine neoplasia type 1 (ref. 15 ), which is an autosomal-dominant syndrome characterized by concurrent parathyroid adenomas, gastroenteropancreatic tumours and several other tumour types. Menin does not share significant amino-acid sequence similarity with other proteins, but it possesses nuclear localization signals within its C terminus [16] . Menin interacts with H3K4 methyltransferases, including mixed-lineage leukaemia 1(MLL1) [17] , and it is an oncogenic cofactor for MLL-associated leukemogenesis [18] , [19] . Also Menin is known to associate with a trithorax family histone methyltransferase complex and contributes to the DNA damage response and cell cycle regulation [20] , [21] . Paradoxically, Menin recruits polycomb repressive complex 2 (PRC2) at the pleiotrophin ( PTN ) locus, and its loss abrogates the binding of the PRC2 components enhancer of zeste homologue 2 (EZH2) and SUZ12 to PTN in lung adenocarcinoma cells [22] . Further, Menin associates with the JunD proto-oncogene product (JUND), nuclear factor of kappa light poly peptide gene enhancer in B cells 1 (NF-κB), peroxisome proliferator-activated receptor gamma (PPAR-γ), SMAD family member 3 (SMAD3) and β-catenin, indicating its involvement in transcriptional activation and repression [23] , [24] . Bach2 (BTB and Cap’n’collar (CNC) homology 1; basic leucine zipper transcription factor 2) belongs to the CNC gene family [25] . B cells preferentially express Bach2, which is critical for somatic hypermutation and class-switch recombination [26] , [27] , and are involved in the IgG1 memory B-cell formation [28] . Bach2 also participates in T-cell-mediated immune responses [29] , [30] , regulates T reg -mediated immune homeostasis and suppresses multiple CD4 T-cell effector programmes [29] . Bach2 -deficient animals suffer from lethal lung and small intestinal inflammation. Bach2 is required for maintaining naive CD4 T cells by suppressing the effector memory-related gene expression [30] . Bach2 deficiency in CD4 T cells reduces the naive CD4 T-cell numbers and enhances the effector memory T cells, particularly T H 2 type. Furthermore, polymorphisms in BACH2 are associated with multiple inflammatory diseases [31] , [32] , [33] . More recently, the involvement of Bach2 in memory CD8 T-cell formation has been reported [34] . These findings establish Bach2 as a key regulator of T-cell-mediated immune homeostasis. In this study, we show that T-cell-specific Menin deficiency induces premature CD4 T-cell senescence, which is accompanied by SASP after antigenic stimulation. Furthermore, Menin-knockout (KO) naive CD4 T cells exhibited a dysregulated production of cytokines. We identify Bach2 as a direct target of Menin that regulates senescence and cytokine production. ChIP sequencing revealed that Menin binds to the Bach2 locus and controls Bach2 expression through the maintenance of histone acetylation. A decreased Menin binding and the Bach2 expression were detected in the senescent CD4 T cells. These findings define a critical role of the Menin-Bach2 pathway in regulating CD4 T-cell-mediated immune homeostasis. Menin deficiency induces CD4 T-cell senescence To determine Menin’s role in CD4 T-cell functions, we crossed Menin flox/flox mice with CD4-Cre transgenic (TG) mice. As previously reported, the T-cell numbers were moderately decreased in the spleen and mesenteric lymph node of Menin flox/flox x CD4-Cre TG (Menin KO) mice ( Supplementary Fig. 1a ) [35] . Menin KO naive CD4 T cells expressed wild-type (WT) levels of interleukin ( Il )- 2 mRNA after T-cell receptor (TCR) stimulation ( Supplementary Fig. 1b ). Il-4 and interferon ( Ifn ) -γ mRNAs were not detected in either WT or Menin KO naive CD4 T cells ( Supplementary Fig. 1b ). The early-phase cell division (days 1–3) induced by TCR stimulation was enhanced in the Menin KO naive CD4 T cells ( Supplementary Fig. 1c ). First, we assessed the role of Menin in CD4 T-cell growth in vitro . Although Menin KO naive CD4 T cells normally expanded after stimulation, the growth rate was reduced after day 4, even in the presence of exogenous IL-2 ( Fig. 1a ). To assess the effects of Menin deficiency on the cell cycle, we measured the percentage of replicating cells after incubation with 5-ethynyl-2′-deoxyuridine (EdU). While approximately 50% of the WT CD4 T cells were EdU positive, indicating replication (S phase), only approximately 30% of Menin KO CD4 T cells were positive 7 days after the initial TCR stimulation ( Fig. 1b ). A reduced number of EdU-positive cells was also detected in the Menin KO CD4 T-cell cultures on days 3 and 5 ( Supplementary Fig. 2a ). Increased expression of cyclin-dependent kinase (CDK) inhibitors, Cdkn1a , Cdkn2a and Cdkn2b , was detected in the Menin KO CD4 T cells ( Fig. 1c ). Cell death was increased in the Menin KO CD4 T-cell cultures (Annexin V positive: approximately 40%) compared with that in WT cultures (Annexin V positive: approximately 20%) ( Fig. 1d ). Increased cell death was detected in the Menin KO CD4 T-cell cultures starting 3 days after the initial stimulation ( Supplementary Fig. 2b ). There was also increased expression of the mRNA encoding pro-apoptotic factors, such as p19 arf , TP53 apoptosis effector (Perp) and phorbol-12-myristate-13-acetate-induced protein 1 (Pmaip1) ( Fig. 1e ), indicating that the reduced number of Menin KO CD4 T cells after day 4 was caused by reduced cell cycle progression and an increased rate of cell death. 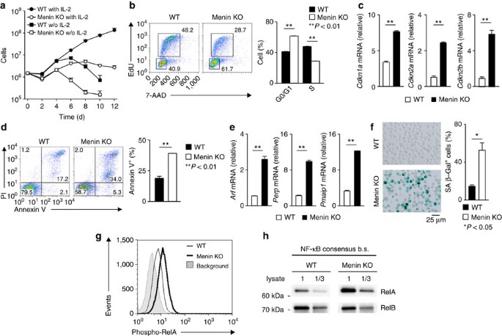Figure 1: Menin deficiency induces premature CD4 T-cell senescence. (a) The TCR-induced proliferation of the Menin KO naive CD4 T cells in the presence or absence of IL-2. The average of three independent cultures and s.d. are shown. (b) The results of the cell cycle analysis of CD4 T cells from the Menin KO and WT mice cultured under IL-2 conditions for 7 days. The percentages of G0/G1- and S-phase cells in three independent cultures are shown (right). (c) The results of the quantitative reverse transcriptase polymerase chain reaction (RT-PCR) analysis of mRNA encodingCdkinhibitors (vertical axes) in the WT and Menin KO THcells. The results represent the expression levels relative toHprtwith the s.d. (d) The results of the cell death analysis of CD4 T cells from the WT and Menin KO mice on day 7. The percentages of annexin V-positive cells in three independent cultures are shown (right). (e) The results of the quantitative RT-PCR analysis of mRNAs encoding pro-apoptotic proteins (vertical axes) in the WT and Menin KO THcells, with the s.d. The results are presented relative to the mRNA expression ofHprtwith the s.d. (f) SA β-galactosidase (SA β-Gal) staining of the THcells from the Menin KO and WT control mice cultured under IL-2-conditions for 7 days (left). The percentages of SA β-Gal-positive cells in three independent cultures with the s.d. are shown (right). (g) The phosphorylation of RelA (Ser534) in the WT and Menin KO THcells cultured for 7 days. (h) Assay of the binding of RelA and RelB to an NF-κB-binding consensus motif in the WT and Menin KO THcells cultured under IL-2 conditions for 7 days. Four (panelcande) and three (panelsa,b,d,f,gandh) independent experiments were performed. *P<0.01, **P<0.01 (Student’st-test). Figure 1: Menin deficiency induces premature CD4 T-cell senescence. ( a ) The TCR-induced proliferation of the Menin KO naive CD4 T cells in the presence or absence of IL-2. The average of three independent cultures and s.d. are shown. ( b ) The results of the cell cycle analysis of CD4 T cells from the Menin KO and WT mice cultured under IL-2 conditions for 7 days. The percentages of G0/G1- and S-phase cells in three independent cultures are shown (right). ( c ) The results of the quantitative reverse transcriptase polymerase chain reaction (RT-PCR) analysis of mRNA encoding Cdk inhibitors (vertical axes) in the WT and Menin KO T H cells. The results represent the expression levels relative to Hprt with the s.d. ( d ) The results of the cell death analysis of CD4 T cells from the WT and Menin KO mice on day 7. The percentages of annexin V-positive cells in three independent cultures are shown (right). ( e ) The results of the quantitative RT-PCR analysis of mRNAs encoding pro-apoptotic proteins (vertical axes) in the WT and Menin KO T H cells, with the s.d. The results are presented relative to the mRNA expression of Hprt with the s.d. ( f ) SA β-galactosidase (SA β-Gal) staining of the T H cells from the Menin KO and WT control mice cultured under IL-2-conditions for 7 days (left). The percentages of SA β-Gal-positive cells in three independent cultures with the s.d. are shown (right). ( g ) The phosphorylation of RelA (Ser534) in the WT and Menin KO T H cells cultured for 7 days. ( h ) Assay of the binding of RelA and RelB to an NF-κB-binding consensus motif in the WT and Menin KO T H cells cultured under IL-2 conditions for 7 days. Four (panel c and e ) and three (panels a , b , d , f , g and h ) independent experiments were performed. * P <0.01, ** P <0.01 (Student’s t -test). Full size image Early cell cycle arrest accompanied by the increased expression of Cdk inhibitors is a hallmark of cellular senescence [8] , suggesting that premature senescence is induced after TCR stimulation of Menin KO CD4 T cells. Although the Menin-deficient naive CD4 T cells did not express a senescence-associated β-galactosidase (SA β-Gal) activity, a maker of cellular senescence, the proportion of SA β-Gal-positive cells was increased in the Menin KO CD4 T-cell cultures 3 days after TCR-mediated stimulation ( Supplementary Fig. 2c ). A strong expression of the SA β-Gal activity was detected in the Menin KO effector CD4 T (T H ) cells on day 7 ( Fig. 1f ). NF-κB signalling induces cellular senescence [36] , [37] , [38] , and the transcription factor NF-κB subunit p65 (RelA) accumulates on the chromatin of senescent cells [39] . In the Menin KO T H cells, enhanced phosphorylation of RelA (pSer534) was detected ( Fig. 1g ) and its DNA-binding activity increased; however, that of the RelB did not increase ( Fig. 1h ), thus indicating that the Menin KO CD4 T cells more rapidly senesced after receiving TCR stimulation than did the WT control cells. The role of Menin in CD4 T response in vivo To investigate the role of Menin in CD4 T-cell expansion and survival in vivo , we monitored antigen-specific CD4 T cells following immunization in an adoptive transfer model. Naive BALB/c mice were transplanted with the Menin KO or WT naïve CD4 T cells and immunized with ovalbumin (OVA) plus lipopolysaccharide (LPS). After 4 days, the number of transplanted Menin KO cells was approximately 25% of that of the WT cells, and the number decreased further on day 7, and the cells did not accumulate in the spleen during the memory phase (day 50) ( Fig. 2a ). 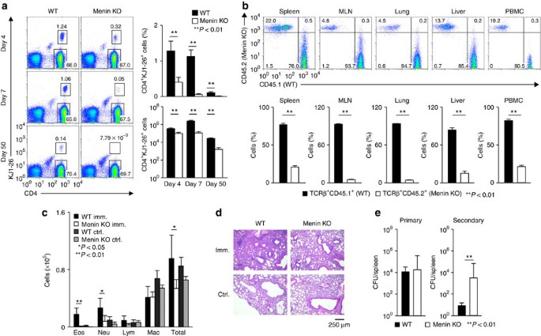Figure 2: Menin is required for the expansion and survival of antigen-stimulated CD4 T cellsin vivo. (a) CD4 T cells from the spleens of the WT or Menin KO mice with a DO11.10 TG background were transferred into syngenic BALB/c mice, and the mice were then immunized with OVA (100 μg) plus LPS (10 μg) (n=5). The transferred OVA-TCR (KJ-1)-positive cells were monitored using FACS on the indicated days. The percentages (upper) and numbers (lower) of KJ1-positive cells are indicated (right). (b) The WT (CD45.1) and Menin KO (CD45.2) THcells were mixed 1:1 and transferred into TCR-βδ KO mice (n=5). Representative staining patterns gated on TCR-β-positive cells (upper) and the percentage (lower) of CD45.1 and CD45.2 cells 4 weeks after transfer are indicated. (c) Quantification of eosinophils (Eos), neutrophils (Neu), lymphocytes (Lym), macrophages (Mac) and total cells in the bronchioalveolar (BAL)-fluid from the WT and Menin KO mice (n=5 per group) that were not immunized (ctrl.) or immunized with OVA plus alum (imm.). (d) The microscopic findings of the lungs from mice as inc, fixed and stained with haematoxylin and eosin. (e) The effects ofMenindeficiency onL. monocytogenes(LM) infection. The bacterial burden in the spleen was determined 3 days after the primary (n=6) and secondary (n=8) infections, respectively. The data represent the findings of three (a,b) or two (c,dande) independent experiments. *P<0.05, **P<0.01 (Student’st-test). Figure 2: Menin is required for the expansion and survival of antigen-stimulated CD4 T cells in vivo . ( a ) CD4 T cells from the spleens of the WT or Menin KO mice with a DO11.10 TG background were transferred into syngenic BALB/c mice, and the mice were then immunized with OVA (100 μg) plus LPS (10 μg) ( n =5). The transferred OVA-TCR (KJ-1)-positive cells were monitored using FACS on the indicated days. The percentages (upper) and numbers (lower) of KJ1-positive cells are indicated (right). ( b ) The WT (CD45.1) and Menin KO (CD45.2) T H cells were mixed 1:1 and transferred into TCR-βδ KO mice ( n =5). Representative staining patterns gated on TCR-β-positive cells (upper) and the percentage (lower) of CD45.1 and CD45.2 cells 4 weeks after transfer are indicated. ( c ) Quantification of eosinophils (Eos), neutrophils (Neu), lymphocytes (Lym), macrophages (Mac) and total cells in the bronchioalveolar (BAL)-fluid from the WT and Menin KO mice ( n =5 per group) that were not immunized (ctrl.) or immunized with OVA plus alum (imm.). ( d ) The microscopic findings of the lungs from mice as in c , fixed and stained with haematoxylin and eosin. ( e ) The effects of Menin deficiency on L. monocytogenes (LM) infection. The bacterial burden in the spleen was determined 3 days after the primary ( n =6) and secondary ( n =8) infections, respectively. The data represent the findings of three ( a , b ) or two ( c , d and e ) independent experiments. * P <0.05, ** P <0.01 (Student’s t -test). Full size image To further examine the role of Menin in the survival of CD4 T cells after antigenic stimulation, in vitro -activated effector CD4 T cells from WT (CD45.1) and Menin KO (CD45.2) mice were mixed 1:1 and adoptively transferred into naive TCR-βδ KO mice. As shown in Fig. 2b , significant reductions of CD45.2-positive Menin KO CD4 T cells were detected in all the tested tissues (the spleen, liver, lung and PBMCs) 4 weeks after the cell transfer. Next, we investigated the airway inflammation in Menin KO mice using an in vivo model. WT and Menin KO mice were immunized with OVA containing alum and then were challenged with inhaled OVA. This decreased the inflammatory cell infiltration in the bronchioalveolar lavage (BAL) fluid of the OVA-immunized Menin KO mice compared with that in WT mice ( Fig. 2c ). The number of mononuclear cells infiltrating the peribronchiolar regions of the lungs in Menin KO mice also decreased ( Fig. 2d ). Finally, we assessed the impact of Menin deficiency on the host defenses against Listeria monocytogenes (Lm) infection. The bacterial burden in the spleens of the Menin KO mice 3 days after primary infection was comparable to that observed in the WT mice ( Fig. 2e , left panel). However, the bacterial burden was significantly higher in the Menin KO mice than in the WT mice after secondary Lm infection (recall response) ( Fig. 2e , right panel). These results indicate that the expansion, survival and function of antigen-stimulated CD4 T cells in vivo require Menin. Menin-deficient CD4 T cells exhibit the SASP phenotype Decreased cell-surface expression of CD27 and CD62L and increased expression of cytotoxic T-lymphocyte-associated protein 4 (CTLA-4) are characteristics of exhausted and senescent T cells [40] , [41] , [42] . The numbers of CD27 low /CD62L low and CD27 high /CD62L low cells were markedly increased in the Menin KO CD4 T-cell cultures compared with those observed in the WT-cell cultures ( Fig. 3a and Supplementary Fig. 3a ). In addition, moderate upregulation of CTLA-4 was detected in the Menin KO T H cells, the level of which was elevated following immobilized anti-TCR-β mAb restimulation ( Supplementary Fig. 3b ). 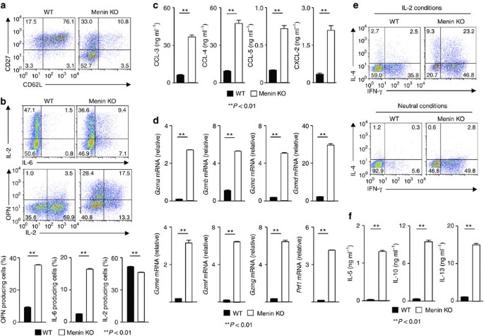Figure 3:Menin-deficient effector CD4 T cells exhibit a senescence-associated secretory phenotype. (a) The staining profile of CD62L/CD27 on the cell surface of the WT and Menin KO THcells. The cell numbers are indicated in each quadrant. (b) The results of the intracellular FACS analysis of IL-2/IL-6, or IL-2/OPN in the WT and Menin KO THcells. The percentages with s.d. of IL-2-, IL-6- and OPN-producing cells in three independent cultures are shown (lower). (c) The ELISA of chemokines in supernatants of the cells inb. (d) The results of the quantitative RT-PCR analysis ofGzm’sandPrf1in cells inb. The results are presented relative to the expression ofHprtmRNA with the s.d. (e) The results of the intracellular FACS analysis of IL-4 and IFN-γ in cells cultured under IL-2- (top) or neutral-conditions (bottom). The numbers of cells are indicated in each quadrant. (f) The ELISA of cytokines in supernatants of the cells cultured under IL-2 conditions and restimulated with an immobilized anti-TCR-β for 16 h. All experiments were performed with THcells cultured under IL-2 conditions for 5 days. At least three independent experiments (a–f) were performed. **P<0.01 (Student’st-test). Figure 3: Menin -deficient effector CD4 T cells exhibit a senescence-associated secretory phenotype. ( a ) The staining profile of CD62L/CD27 on the cell surface of the WT and Menin KO T H cells. The cell numbers are indicated in each quadrant. ( b ) The results of the intracellular FACS analysis of IL-2/IL-6, or IL-2/OPN in the WT and Menin KO T H cells. The percentages with s.d. of IL-2-, IL-6- and OPN-producing cells in three independent cultures are shown (lower). ( c ) The ELISA of chemokines in supernatants of the cells in b . ( d ) The results of the quantitative RT-PCR analysis of Gzm’s and Prf1 in cells in b . The results are presented relative to the expression of Hprt mRNA with the s.d. ( e ) The results of the intracellular FACS analysis of IL-4 and IFN-γ in cells cultured under IL-2- (top) or neutral-conditions (bottom). The numbers of cells are indicated in each quadrant. ( f ) The ELISA of cytokines in supernatants of the cells cultured under IL-2 conditions and restimulated with an immobilized anti-TCR-β for 16 h. All experiments were performed with T H cells cultured under IL-2 conditions for 5 days. At least three independent experiments ( a – f ) were performed. ** P <0.01 (Student’s t -test). Full size image The SASP phenotype is characterized by the secretion of pro-inflammatory factors, including IL-6, IL-8 and pro-inflammatory chemokines [10] , [11] , and senescent CD4 T cells produce a high level of osteopontin (OPN) [43] . We found that the number of IL-6- and OPN-producing cells markedly increased in the Menin KO CD4 T-cell cultures, while the number of IL-2-producing cells was marginally decreased ( Fig. 3b ). Increased production of IL-6 and OPN in the Menin KO T H cells was detected using enzyme-linked immunosorbent assays (ELISAs) ( Supplementary Fig. 3c ). The production of pro-inflammatory chemokines, chemokine (C-C motif) ligand 3 (CCL-3), CCL-4, CCL-5 and chemokine (C-X-C motif) ligand 2 (CXCL-2), increased in the Menin KO T H cells ( Fig. 3c ). Using a DNA microarray analysis, we found that the expression of a series of pro-inflammatory factors was upregulated in the Menin KO T H cells compared with that in the WT cells ( Supplementary Data 1 ). For example, the expression of genes encoding the components of cytotoxic granules ( Gzm a , b , c , d , e , f , g, and Prf1 ), which are involved in age-related cardiovascular and pulmonary diseases [44] , markedly increased ( Fig. 3d ). The augmented expression of pro-inflammatory enzymes such as Adam8 , Alox5 , Casp1 , Ctsd and Ctsh was detected in the Menin KO T H cells ( Supplementary Fig. 3d ). The increased production of pro-angiogenic factors is another hallmark of SASP in senescent cells [10] , [45] . The expression of genes encoding pro-angiogenic factors, such as Esm1 , Pdgfα , S100a4 and Vegfc , upregulated in the Menin KO T H cells ( Supplementary Fig. 3e ). These results strongly suggest that Menin deficiency causes the SASP in the effector CD4 T cells. Cytokine productions in Menin-deficient CD4 T cells Changes in the cytokine production profile of senescent CD4 T cells have been previously reported [46] . Next, we analysed the cytokine productions in Menin KO effector CD4 T cell in vitro . The generation of IFN-γ- and IL-4-producing cells was increased in the Menin KO naive CD4 T cell cultured under IL-2 conditions compared with that observed in the WT cells ( Fig. 3e upper panel and Supplementary Fig. 4a ). Furthermore, IL-4/IFN-γ-double producers were induced in Menin KO CD4 T-cell cultures (23.2%) but not in WT cultures (2.5%) ( Fig. 3e upper panel and Supplementary Fig. 4a ). Enhanced generation of IFN-γ-producing cells was detected even in the presence of an anti-IFN-γ mAb, whereas the generation of IL-4-producing cells was blocked by an IL-4-neutralizing antibody ( Fig. 3e lower panel, Supplementary Fig. 4a,b ). The production of T H 2-related cytokines, such as IL-5, IL-10, and IL-13, was increased in the Menin KO T H cells ( Fig. 3f ), while the IL-9, IL-17A and tumour necrosis factor (TNF)-α production levels remained unaffected under IL-2 conditions ( Supplementary Fig. 4c ). To assess the responsiveness of the Menin KO naive CD4 T cells to IL-4 and IL-12, we stimulated naive CD4 T cells with anti-TCR-β and anti-CD28 Ab in the presence of various doses of IL-4 or IL-12. As we previously reported [35] , the Menin-deficient CD4 T cells normally differentiated into IL-4-producing cells under optimal T H 2 culture conditions ( Supplementary Fig. 4d , right panel). Compared with WT cells, the Menin KO naive CD4 T cells readily differentiated into IL-4-producing cells in response to low concentrations of IL-4 ( Supplementary Fig. 4d ). Enhanced generation of IFN-γ-producing cells was detected in the Menin KO CD4 T cells even in the presence of IL-4 ( Supplementary Fig. 4d ). The IL-12-dependent induction of IFN-γ-producing cells was augmented in the Menin KO naïve CD4 T-cell cultures, although the Menin-deficient CD4 T cells normally differentiated into IFN-γ-producing cells under optimal T H 1 culture conditions ( Supplementary Fig. 4e ). These results indicate the crucial role of Menin in regulating the IFN-γ and T H 2 cytokine production in CD4 T cells under the condition with limited concentration of IL-4 or IL-12, respectively. Bach2 is a downstream target of Menin Next, we investigated the molecular mechanisms involved in the induction of SASP and cytokine production in the Menin-deficient cells. On the basis of the results of the DNA microarray analysis, we focused on Bach2 , which was differentially expressed in the Menin KO T H cells ( Supplementary Data 1 ). The Bach2 mRNA ( Fig. 4a , right) and protein levels ( Fig. 4b ) were significantly reduced in the Menin KO T H cells compared with those in the WT cells. The Bach2 mRNA level in the Menin KO naive CD4 T cells was marginally reduced ( Fig. 4a , left). Next, we transduced Bach2 into the Menin KO T H cells. The Bach2 protein levels in the Bach2 -transduced T H cells were comparable to those observed in the WT T H cells ( Supplementary Fig. 5a ). The induction of IL-4- and IFN-γ-producing cells from the Menin KO naïve CD4 T cells was normalized by the transduction of Bach2 ( Fig. 4c , upper panel). The generation of IL-6-producing cells from the Menin KO naive CD4 T cells was also suppressed by the transduction of Bach2 ( Fig. 4c , lower panel). Reduced production of IL-5, IL-10, IL-13 and OPN in the Bach2 -transduced Menin T H cells was detected using ELISAs ( Fig. 4d ). The augmentation of CCL-3, CCL-4, CCL-5 and CXCL-2 in the Menin KO T H cells was also normalized by the Bach2 transduction ( Fig. 4e ). The transduction of the Menin KO T H cells with Bach2 restored the enhanced mRNA expression levels of Gzm’s and Prf1 ( Fig. 4f ), Ctla4 ( Supplementary Fig. 5b ) and the genes that encode pro-inflammatory enzymes and pro-angiogenic factors ( Supplementary Fig. 5c ). 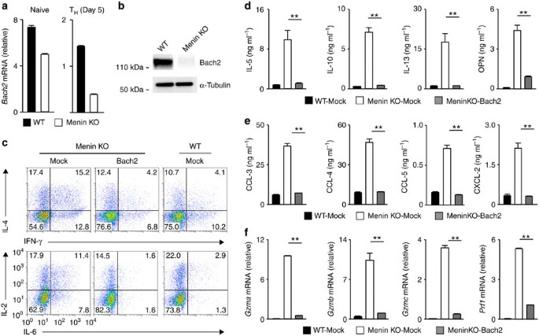Figure 4: Enforced expression ofBach2restores the phenotypes of the Menin KO effector CD4 T cells. (a) The results of the quantitative RT-PCR analysis of mRNA encodingBach2in the WT and Menin KO naive CD4 T (right) and TH(left). The results are presented relative to the mRNA expression ofHprtwith the s.d. (b) The results of the immunoblot analysis of Bach2 in the nuclear fractions of the WT and Menin KO THcells. (c) The results of the intracellular FACS analysis of IL-4/IFN-γ and IL-2/IL-6 in the Menin KO THcells transduced with an empty vector (Mock) or with Bach2-expressing retroviral vector (Bach2). The naive CD4 T cells cultured under IL-2-conditions were infected with retroviral vectors and cultured for 3 days in the presence of IL-2. (d) The mock- or Bach2-transduced cells incwere purified using an AutoMACS device and restimulated with immobilized anti-TCR-β for 16 h. The amounts of cytokines in the supernatants were determined using ELISA. (e) The amounts of pro-inflammatory chemokines in the supernatants indwere determined using ELISA. (f) The results of the quantitative RT-PCR analysis of theGzm’sandPrf1of cells ind. The results are presented relative to the mRNA expression ofHprtwith the s.d. All experiments were performed with THcells cultured under IL-2 conditions for 5 days. Three independent experiments (a–f) were performed. **P<0.01 (Student’st-test). Figure 4: Enforced expression of Bach2 restores the phenotypes of the Menin KO effector CD4 T cells. ( a ) The results of the quantitative RT-PCR analysis of mRNA encoding Bach2 in the WT and Menin KO naive CD4 T (right) and T H (left). The results are presented relative to the mRNA expression of Hprt with the s.d. ( b ) The results of the immunoblot analysis of Bach2 in the nuclear fractions of the WT and Menin KO T H cells. ( c ) The results of the intracellular FACS analysis of IL-4/IFN-γ and IL-2/IL-6 in the Menin KO T H cells transduced with an empty vector (Mock) or with Bach2-expressing retroviral vector (Bach2). The naive CD4 T cells cultured under IL-2-conditions were infected with retroviral vectors and cultured for 3 days in the presence of IL-2. ( d ) The mock- or Bach2-transduced cells in c were purified using an AutoMACS device and restimulated with immobilized anti-TCR-β for 16 h. The amounts of cytokines in the supernatants were determined using ELISA. ( e ) The amounts of pro-inflammatory chemokines in the supernatants in d were determined using ELISA. ( f ) The results of the quantitative RT-PCR analysis of the Gzm’s and Prf1 of cells in d . The results are presented relative to the mRNA expression of Hprt with the s.d. All experiments were performed with T H cells cultured under IL-2 conditions for 5 days. Three independent experiments ( a – f ) were performed. ** P <0.01 (Student’s t -test). Full size image We crossed Bach2 flox/flox mice [28] with CD4-Cre TG mice and generated T-cell-specific Bach2 -deficient (Bach2 KO) mice to confirm the roles of Bach2 in CD4 T-cell senescence and cytokine production. Although the number of T cells was moderately reduced ( Supplementary Fig. 6a ), a significant number of naive CD4 T cells remained in the spleens of the Bach2 KO mice ( Supplementary Fig. 6b ). The generation of IL-4- and IFN-γ-producing cells was accelerated, and IL-4/IFN-γ-double producers were generated in the Bach2 KO naïve CD4 T cells cultured under IL-2 conditions ( Fig. 5a , upper panel). The augmentation of IL-6-producing cells was observed in Bach2 KO T H cells ( Fig. 5a , lower). The levels of IL-5, IL-10, IL-13, OPN and pro-inflammatory chemokines were increased in the Bach2 KO T H cells compared with those in WT cells ( Fig. 5b ). Moreover, the enhanced expression of Gzm’s and Prf1 ( Fig. 5c ), pro-inflammatory factors ( Supplementary Fig. 7a ) and pro-angiogenic factors ( Supplementary Fig. 7b ) was detected in Bach2 KO T H cells. The mRNA for Ctla4 was also upregulated in the Bach2 KO T H cells ( Supplementary Fig. 7c ). The expression of the SA β-Gal activity was increased in the Bach2 KO T H cells ( Fig. 5d ). Furthermore, the DNA-binding activity of RelA was upregulated in the Bach2 KO T H cells ( Fig. 5e ). These data indicate that the senescent phenotypes of Bach2 KO T H cells are similar to those of Menin KO cells. 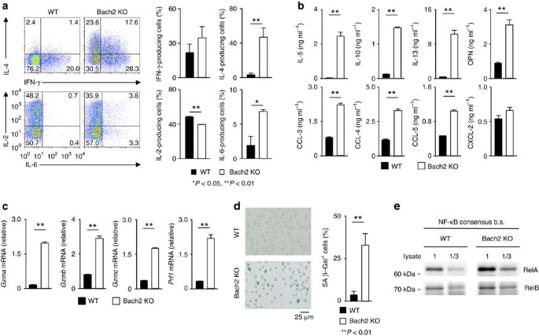Figure 5: Early induction of cellular senescence in the Bach2 KO naive CD4 T cells. (a) The results of the intracellular FACS analysis of IL-4/IFN-γ and IL-2/IL-6 in the Bach2 KO naive CD4 T cells cultured under IL-2-conditions for 7 days. The percentages with the s.d. of IFN-γ-, IL-2-, IL-4- and IL-6- producing cells in three independent cultures are shown (right). (b) The ELISA of cytokines and chemokines in the supernatants of the cells inarestimulated with immobilized anti-TCR-β for 16 h. (c) The results of the quantitative RT-PCR analysis of theGzm’sandPrf1of the cells ina. The results are presented relative to the mRNA expression ofHprtwith the s.d. (d) SA β-galactosidase (SA β-Gal) staining of THcells obtained from Bach2 KO and WT control mice cultured under IL-2-conditions for 10 days (left). The percentages with the s.d. of SA β-Gal-positive cells in three independent cultures are shown (right). (e) Assay of the binding of RelA and RelB to an NF-κB-binding consensus motif in the WT and Bach2 KO THcells. The experiment was performed with THcells cultured under IL-2 conditions for 5 days. Three independent experiments (a–e) were performed. *P<0.05, **P<0.01 (Student’st-test). Figure 5: Early induction of cellular senescence in the Bach2 KO naive CD4 T cells. ( a ) The results of the intracellular FACS analysis of IL-4/IFN-γ and IL-2/IL-6 in the Bach2 KO naive CD4 T cells cultured under IL-2-conditions for 7 days. The percentages with the s.d. of IFN-γ-, IL-2-, IL-4- and IL-6- producing cells in three independent cultures are shown (right). ( b ) The ELISA of cytokines and chemokines in the supernatants of the cells in a restimulated with immobilized anti-TCR-β for 16 h. ( c ) The results of the quantitative RT-PCR analysis of the Gzm’s and Prf1 of the cells in a . The results are presented relative to the mRNA expression of Hprt with the s.d. ( d ) SA β-galactosidase (SA β-Gal) staining of T H cells obtained from Bach2 KO and WT control mice cultured under IL-2-conditions for 10 days (left). The percentages with the s.d. of SA β-Gal-positive cells in three independent cultures are shown (right). ( e ) Assay of the binding of RelA and RelB to an NF-κB-binding consensus motif in the WT and Bach2 KO T H cells. The experiment was performed with T H cells cultured under IL-2 conditions for 5 days. Three independent experiments ( a – e ) were performed. * P <0.05, ** P <0.01 (Student’s t -test). Full size image Menin maintains histone acetylation at the Bach2 locus To investigate the molecular mechanism by which Menin controls the Bach2 expression, we assessed changes in the histone modification of Bach2 in the Menin KO T H cells using a ChIP-seq analysis. The level of H3K4me3 at Bach2 peaked at the transcriptional start site (Tss) and was slightly decreased in the Menin KO T H compared with that in the WT T H cells ( Fig. 6a , upper). The level of H3K27me3 at the Tss of Bach2 was increased in the Menin KO T H cells ( Fig. 6a , middle). Furthermore, the level of acetylated (ac) histone H3K27 was markedly reduced in the Menin KO T H cells ( Fig. 6a , lower). We further compared the histone modifications around the Tss of Bach2 between Menin KO and WT CD4 T cells. A schematic representation of the region surrounding the Tss of Bach2 and the location of the amplicons used in ChIP-qPCR are shown in Supplementary Fig. 8a . Decreased levels of H3K4me3 and H3K27ac and an increased level of H3K27me3 around the Tss of Bach2 were detected in the Menin KO T H cells cultured under IL-2 conditions for 5 days ( Fig. 6b ). Interestingly, a striking reduction in the H3K27ac level was detected in the Menin KO T H -cell cultured for 3 days, while the H3K4me3 level remained unchanged ( Supplementary Fig. 8b ). The level of H3K4me3 was also unaffected in the Menin KO naive CD4 T cells ( Supplementary Fig. 8b ). In addition, we were able to detect only a small reduction in the H3K27ac level, as well as upregulation of H3K27me3, in the Menin KO naive CD4 T cells. ( Supplementary Fig. 8b ). These results suggest that the reduction of H3K27ac observed after TCR stimulation has the primary effect of inducing Menin deficiency. 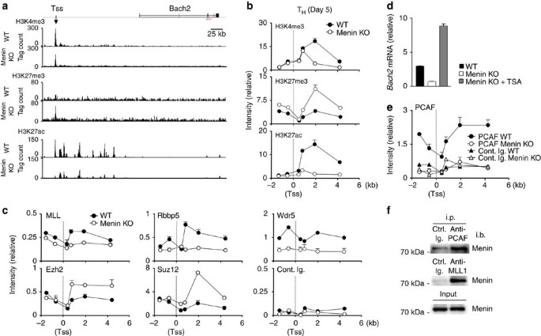Figure 6: Menin controls the Bach2 expression by maintaining the histone acetylation at theBach2locus. (a) The global patterns of histones, H3K4me3 (upper), H3K27me3 (middle) and H3K27ac (lower) at theBach2locus in the WT and Menin KO THcells cultured under IL-2 conditions for 5 days were determined using ChIP-seq. (b) The results of the ChIP assay with a quantitative PCR analysis of the histone modification (H3K4me3, H3K27me3 and H3K27ac) status around the Tss of theBach2locus in the WT and Menin KO THcells. The relative intensity (input) with the s.d. is shown. (c) ChIP with a quantitative PCR analysis of the binding of HMT2A/B (MLL1, Rbbp5 and Wdr5) and PRC2 (Ezh2 and Suz12) components to theBach2Tss region in the Menin KO THcells. (d) The results of the quantitative RT-PCR analysis ofBach2mRNA expression in the Menin KO THcells treated with TSA for 24 h. The results are presented relative to the mRNA expression ofHprtmRNA with the s.d. (e) The ChIP data with the results of the quantitative PCR analysis of PCAF binding to theBach2Tss region. The relative intensity (/input) with the s.d. is shown. (f) The association between Menin and PCAF in the THcells. The nuclear lysates (5 × 106cells) were precipitated with anti-PCAF mAb or anti-MLL1 pAb, and immunoblotted with anti-Menin pAb. Two (a) and three (b–f) independent experiments were performed. **P<0.01 (Student’st-test). All experiments were performed with THcells cultured under IL-2 conditions for 5 days. Figure 6: Menin controls the Bach2 expression by maintaining the histone acetylation at the Bach2 locus. ( a ) The global patterns of histones, H3K4me3 (upper), H3K27me3 (middle) and H3K27ac (lower) at the Bach2 locus in the WT and Menin KO T H cells cultured under IL-2 conditions for 5 days were determined using ChIP-seq. ( b ) The results of the ChIP assay with a quantitative PCR analysis of the histone modification (H3K4me3, H3K27me3 and H3K27ac) status around the Tss of the Bach2 locus in the WT and Menin KO T H cells. The relative intensity (input) with the s.d. is shown. ( c ) ChIP with a quantitative PCR analysis of the binding of HMT2A/B (MLL1, Rbbp5 and Wdr5) and PRC2 (Ezh2 and Suz12) components to the Bach2 Tss region in the Menin KO T H cells. ( d ) The results of the quantitative RT-PCR analysis of Bach2 mRNA expression in the Menin KO T H cells treated with TSA for 24 h. The results are presented relative to the mRNA expression of Hprt mRNA with the s.d. ( e ) The ChIP data with the results of the quantitative PCR analysis of PCAF binding to the Bach2 Tss region. The relative intensity (/input) with the s.d. is shown. ( f ) The association between Menin and PCAF in the T H cells. The nuclear lysates (5 × 10 6 cells) were precipitated with anti-PCAF mAb or anti-MLL1 pAb, and immunoblotted with anti-Menin pAb. Two ( a ) and three ( b – f ) independent experiments were performed. ** P <0.01 (Student’s t -test). All experiments were performed with T H cells cultured under IL-2 conditions for 5 days. Full size image Menin is a component of the KMT2A/2B complex, which is involved in the methylation of histone H3K4, an active histone marker [17] . We assessed changes in the binding of KMT2A/2B and PRC2 components at Bach2 in the Menin KO T H cells using ChIP-qPCR. As shown in Fig. 6c , the binding of the KMT2A/2B complex, including that with MLL1, Rbbp5 and Wdr5, was decreased in the Menin KO T H cells, whereas the binding of Ezh2 and Suz12 (PRC components) was augmented ( Fig. 6c ). However, the level of binding of the KMT2A/2B complex with the Bach2 gene was relatively low. Next, we treated Menin KO T H cells with trichostatin A (TSA), an HDAC inhibitor, to determine the role of histone acetylation in maintaining Bach2 transcription. The Bach2 expression in the Menin KO T H cells was completely restored by TSA treatment ( Fig. 6d ). The recruitment of RNA polymerase II and the H3K4me3 and H3K27ac status at the Tss of the Bach2 gene locus were also restored by TSA ( Supplementary Fig. 8c ). We detected enhanced binding of HDAC1 at the Bach2 locus in the Menin KO mice, and the level of which was reduced by TSA treatment ( Supplementary Fig. 8d ). To identify histone acetyltransferases that are recruited in a Menin-dependent manner, we performed a series of ChIP-qPCR assays and found that the binding of lysine acetyltransferase 2B (PCAF) around the Bach2 Tss was reduced in the Menin KO T H cells ( Fig. 6e ). The binding of other HATs, such as CBP and p300, to the Bach2 Tss in the Menin KO T H cells was comparable to that observed in the WT T H cells ( Supplementary Fig. 8e ). In addition, the physical association between PCAF and Menin was detected in the WT T H cells ( Fig. 6f ). These results suggest that the primary result of Menin deficiency is the inability to maintain active histone modification at the Bach2 locus after TCR stimulation. Menin controls Bach2 expression in the senescent T H cells To determine whether the expression of Menin and/or Bach2 is reduced in senescent CD4 T cells, we established a senescent T H (sT H ) cell induction model ( Supplementary Fig. 9a ). The CD62L low /CD27 high and CD62L low /CD27 low populations were increased in the sT H culture in comparison with that observed in the primary effector CD4 T cells (pT H ) culture ( Supplementary Fig. 9b ). The number of IL-6-, IL-10- and OPN-producing cells was also increased in the sT H cultures that observed in the pT H culture ( Supplementary Fig. 9c ). Therefore, we concluded that sT H have senescent CD4 T-cell-like characteristics. The mRNA and protein expressions of Bach2 in the sT H cells were lower than those observed in the pT H cells ( Fig. 7a,b ). In sharp contrast, the expression of Menin in the sT H cells was comparable to that observed in the pT H cells ( Fig. 7a,b ). Next, we performed ChIP sequencing using an anti-Menin antibody to compare the binding levels of Menin at the Bach2 locus in the sT H and in pT H cells. As shown in Fig. 7c , Menin binding was detected around the Tss of the Bach2 gene, spread towards the 3′ sites in the pT H cells. The level of Menin binding was decreased in the sT H cells, and a reduction in the H3K4me3 and H3K27ac levels was also detected at the Bach2 in the sT H cells ( Fig. 7d ). The decreased binding of Menin around the Tss at the Bach2 gene locus was confirmed using ChIP-qPCR. A reduction in the binding of RNA polymerase II (PNAPII), PCAF, MLL1, Rbbp5 and Wdr5, as well as an increase in the binding of Suz12 at the Bach2 was also detected in the sT H cells ( Fig. 7e ). Although the reduced expression of Bach2 mRNA ( Fig. 7d ) and the level of H3K27ac ( Supplementary Fig. 9d ) in the sT H cells were completely restored by TSA treatment ( Fig. 7f ), the recruitment of Menin at the Bach2 locus was not increased in the TSA-treated sT H cells ( Supplementary Fig. 9e ). These results indicate that the Menin-dependent maintenance of histone acetylation is required for the proper expression of Bach2 , whereas Menin is not essential for Bach2 transcription. 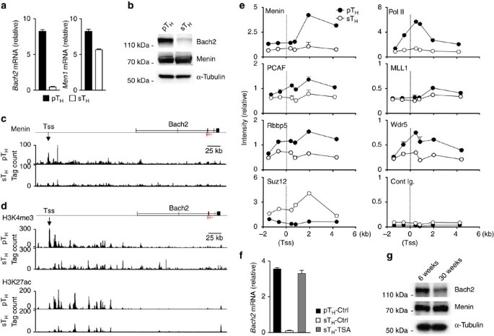Figure 7: Menin is involved in the regulation of theBach2gene expression in senescent CD4 T cells. (a) A quantitative RT-PCR analysis of theBach2andMeninmRNA expression in senescent effector CD4 T (sTH) cells. The results are presented relative to the expression ofHprtmRNA with the s.d. (b) An immunoblot analysis of Bach2 and Menin in the nuclear fractions of the primary effector CD4 T (pTH) and sTHcells. The α-tubulin proteins in the cytosolic fractions were blotted as a loading control. (c) The global patterns of Menin binding at theBach2gene locus in the pTHand sTHcells were determined using ChIP sequencing. (d) The global patterns of histones H3K4me3 and H3K27ac at theBach2gene locus in the pTHand sTHcells were determined using ChIP sequencing. (e) ChIP with quantitative PCR analysis of Menin, RNA polymerase II, KMT2A/2B components and Suz12 in the pTHand sTHcells. The relative intensity (input) is shown with the s.d. (f) A quantitative RT-PCR analysis of theBach2mRNA expression in the sTHcells treated with TSA for 24 h. The results are presented relative to the expression ofHprtmRNA with the s.d. (g) A decreased Bach2 protein expression in the elderly THcells. Bach2 protein expression in young (6 weeks old) and elderly (30 week old) was determined by immunoblotting. Three (a,b,e,fandg) and two (c,d) independent experiments were performed with similar results. **P<0.01 (Student’st-test). Figure 7: Menin is involved in the regulation of the Bach2 gene expression in senescent CD4 T cells. ( a ) A quantitative RT-PCR analysis of the Bach2 and Menin mRNA expression in senescent effector CD4 T (sT H ) cells. The results are presented relative to the expression of Hprt mRNA with the s.d. ( b ) An immunoblot analysis of Bach2 and Menin in the nuclear fractions of the primary effector CD4 T (pT H ) and sT H cells. The α-tubulin proteins in the cytosolic fractions were blotted as a loading control. ( c ) The global patterns of Menin binding at the Bach2 gene locus in the pT H and sT H cells were determined using ChIP sequencing. ( d ) The global patterns of histones H3K4me3 and H3K27ac at the Bach2 gene locus in the pT H and sT H cells were determined using ChIP sequencing. ( e ) ChIP with quantitative PCR analysis of Menin, RNA polymerase II, KMT2A/2B components and Suz12 in the pT H and sT H cells. The relative intensity (input) is shown with the s.d. ( f ) A quantitative RT-PCR analysis of the Bach2 mRNA expression in the sT H cells treated with TSA for 24 h. The results are presented relative to the expression of Hprt mRNA with the s.d. ( g ) A decreased Bach2 protein expression in the elderly T H cells. Bach2 protein expression in young (6 weeks old) and elderly (30 week old) was determined by immunoblotting. Three ( a , b , e , f and g ) and two ( c , d ) independent experiments were performed with similar results. ** P <0.01 (Student’s t -test). Full size image Finally, we compared the expression levels of Bach2 in T H cells obtained from young and elderly mice. As shown in Fig. 7g , the Bach2 expression was lower in the elderly T H cells than in the young T H cells. In addition, a substantial number of elderly T H cells rapidly expressed an SA β-Gal activity ( Supplementary Fig. 10 ). These results demonstrate a correlation between ageing and the Bach2 expression. In this study, we demonstrated the critical role that the Menin-Bach2 pathway plays in regulating CD4 T-cell senescence and cytokine production. Menin KO T H cells exhibited phenotypes that are characteristics of cellular senescence, including a reduced growth rate, increased SA β-Gal activity, prolonged activation of p65/RelA and induction of SASP after TCR stimulation. Furthermore, the generation of IL-4- and IFN-γ-producing cells was augmented in the Menin KO naive CD4 T cells in particular under IL-2 culture conditions. The transcription repressor Bach2, which inhibits senescence and abnormalities in cytokine production, was identified to be a downstream target of Menin. The transduction of Bach2 into the Menin KO T H cells restored the SASP and cytokine production. In contrast, the Bach2 KO CD4 T cells rapidly expressed a senescent phenotype following TCR stimulation, with an increase in the generation of IL-4- and IFN-γ-producing cells in particular under IL-2 culture conditions. The decreased binding of Menin around Tss at the Bach2 gene and a reduction in the Bach2 expression were detected in the artificially induced senescent T H (sT H ) cells. We thus concluded that the Menin-Bach2 axis represses the transcriptional programme that controls cellular senescence and cytokine production and is involved in immunosenescence. CD4 T cells play an essential role in mediating humoral and cellular immune responses. Therefore, the age-associated dysfunction of CD4 T cells has a strong impact on the immune system. Our present study revealed the important role of the Menin-Bach2 pathway in regulating CD4 T-cell homeostasis. BACH2 polymorphisms are associated with multiple inflammatory diseases in humans [31] , [32] , [33] . Bach2 regulates process of immune homeostasis dependent on T reg and multiple effector programmes in CD4 T cells, and the spontaneous onset of lethal lung and small intestinal inflammation occurs in Bach2 -null animals [29] . We observed an augmentation of the generation of IFN-γ− and T H 2 cytokine-producing cells in the Bach2 KO naive CD4 T-cell cultures. Taken together, these data suggest that the Menin-Bach2 axis regulates CD4 T-cell immune homeostasis and protects against the onset of multiple inflammatory disorders. Although Bach2 plays a crucial role in T-cell-mediated immune responses [29] , [30] , the mechanism regulating its physiological expression is unknown. Our present study reveals the crucial role of Menin in the regulation of Bach2 expression in CD4 T cells. However, Menin may not be essential for Bach2 transcription, because the mRNA expression of Bach2 was only minimally reduced in the Menin -deficient naive CD4 T cells. Several studies have indicated that Menin is involved in the regulation of gene transcription through histone modifications [47] , [48] , [49] . Menin interacts with histone methyltransferases MLL1 (ref. 17 ) to regulate transcription. The Menin-MLL histone methyltransferase complex contains other components encoded by Ash2l , Rbbp5 and Wdr5 ; however, the molecules do not always co-localize with Menin [50] . Moreover, it has been reported that Menin and MLL1 regulate distinct pathways during normal haematopoiesis and B-cell development [51] . We herein demonstrated that the primary effect of Menin deficiency was to reduce the H3K27ac, but not H3K4me3, levels at the Bach2 locus. The binding of the histone acetyltransferase, PCAF, at the Bach2 locus was decreased in the Menin KO T H cells. These results suggest that Menin forms complexes with PCAF that have not yet been identified and preserves the Bach2 expression in CD4 T cells by maintaining H3K27 acetylation. This was further indicated by the finding that TSA treatment restored the Bach2 expression in the Menin KO T H cells. In contrast, we were unable to detect Bach2 proteins in the Menin KO T H cells using immunoblotting, whereas a considerable amount of Bach2 mRNA continue to be expressed. Therefore, Menin may regulate the Bach2 expression via both transcriptional and post-transcriptional mechanism, thereby controlling CD4 T senescence and cytokine homeostasis during CD4 T-cell activation. A recent report indicated that Menin has modest effects on haematopoiesis under steady-state conditions, while playing a crucial role in the long-term maintenance of haematopoietic stem cells (HSCs), particularly under conditions of haematopoietic stress [52] . A significant decrease in the number of B cells was observed in the tamoxifen-administered Menin flox/flox x CreER TG mice, and a mixed bone marrow transfer assay revealed a cell-autonomous reduction in the generation of myeloid, B and T cells from Menin -deleted HSCs [52] . We found that the number of mature T cells was modestly decreased in the spleens of the Menin flox/flox x CD4 - Cre TG mice. In addition, the number of Menin-deficient CD4 T cells further decreased after TCR stimulation. The present study indicates that Menin maintains the number of CD4 T cells in part by inhibiting cellular senescence. It is possible that Menin also plays a crucial role in inhibiting the senescence of HSCs induced by haematopoietic stress and is therefore required for the long-term maintenance of HSCs. Menin regulates haematopoiesis in part by regulating the Hox gene expression [19] . However, we were unable to detect a reduced Hox gene expression in the Menin KO T H cells using a DNA microarray analysis. Therefore, Menin presumably regulates CD4 T-cell senescence and cytokine production in a Hox-independent manner. We detected prolonged activation of NF-kB p65 (RelA) in the Menin KO T H cells. The low level and prolonged activation of RelA is a common characteristic of senescent cells [8] , [11] , and RelA accumulates on the chromatin of senescent cells and acts as a master regulator of the SASP [39] . Menin interacts with the NF-kB components both in vitro and in vivo , and represses the transcriptional activation of an NF-kB reporter gene stimulated by phorbol-12-myristate-13-acetate or TNF-α [24] . Moreover, prolonged activation of RelA was also detected in the Bach2 KO T H cells. Therefore, Menin modulates the NF-κB-dependent signalling pathway in CD4 T cells via multiple pathways, thereby regulating the NF-kB-mediated induction of the age-dependent gene expression and senescence. In conclusion, we herein demonstrated that Menin controls cellular senescence and cytokine production, and it is involved in the fate decision of CD4 T cells after TCR-mediated activation. Bach2 acts downstream of Menin in the regulation of the senescence and cytokine production. These findings revealed that Menin controls CD4 T-cell-mediated immune homeostasis, at least in part, by regulating the expression of Bach2. Moreover, Bach1, a homologue of Bach2, repressed the oxidative stress-induced cellular senescence of MEF [53] . Taken together, the data presented here indicate that Bach repressors may play a crucial role in repressing cellular senescence and in the subsequent age-associated development of various disorders, such as cancer and inflammatory diseases. Mice Menin flox/flox mice, TCR-βδ KO mice and Cre TG mice under the control of the Cd4 promoter were purchased from The Jackson Laboratory. Menin flox/flox × CD4 Cre Tg mice with BALB/c mice were generated by Dr Toshinori Nakayama (Chiba University, Chiba, Japan). Bach2 flox/flox mice were established by Dr Tomohiro Kurosaki (RIKEN and Osaka University) [28] , OVA-specific αβTCR (DO11.10) TG mice were provided by Dr D. Loh (Washington University School of Medicine, St Louis, USA) [54] , and C57BL/6 and BALB/c mice were purchased from Clea (Clea Japan, Tokyo, Japan). The female mice were used in in vivo experiments. For in vitro experiments, both male and female mice were used. All mice were maintained under specific pathogen-free conditions and were then used at 6-10 weeks of age. All experiments using mice received approval from the Kazusa DNA Research Institute and Ehime University Administrative Panel for Animal Care. All animal care was conducted in accordance with the guidelines of the Kazusa DNA Research Institute and Ehime University. Antibodies Antibodies used for intracellular and cell-surface staining were as follows: anti-IL-4-phycoerythrin (PE) mAb (11B11; BD Bioscience), IFN-γ-FITC mAb (XMG1.2; BD Bioscience), IL-5-allophycocyanin (APC) (TRFK5; eBioscience), IL-13-PE (eBio13A; eBioscience), IL-2-APC mAb (JES6-5H4; eBioscience), IL-6-PE (MP5-20F3; BioLegend), IL-9-PE (RM9A4; BioLegend), IL-10-APC (JES5-16E3; BD Biosciences), IL-17A-PE (TC11-18H10.1; BioLegend), OPN-PE (cat#IC808P; R&D systems), Foxp3-Alexa Fluor 647 (150D; BioLegend) and NF-κB p65-Alexa Fluor 647 (cat#448; Cell Signaling Technology), CD27-PE (LG.7F9; eBioscience), CD62L-APC (MEL-14; BD Biosciences), CTLA-4 (CD152) -PE (UC10-4B9; eBioscience) and anti-TCR DO11.10-PE (KJ1-26; BioLegend). Antibodies for immunoblotting were as follows: anti-Menin pAb (cat#A300-105A; Bethyl Laboratories), anti-Bach2 pAb (cat#SAB2100201; Thermo Scientific), anti-NF-κB p65 mAb (cat#8242; Cell Signaling Technology), anti-RelB pAb (sc-226; Santa Cruz Biotechnology) and anti-α-tubulin mAb (cat#MS-581-P; NeoMarkers). Antibodies used for ChIP assay were as follows: anti-histone H3K4me3 pAb (cat#39159; Active Motif), anti-histone H3K27ac pAb (cat#39133; Active Motif), anti-histone H3K27me3 pAb (cat#39155; Active Motif), anti-Menin pAb (cat#A300-105A; Bethyl Laboratories), anti-Bach2 ant-serum (cat#SAB2100201; Thermo Scientific), anti-RNA polymerase II mAb (8WG16 cat#05-952; MERCK MILLIPORE), anti-PCAF mAb (cat#3378; Cell Signaling Technology), anti-MLL pAb (cat#A300-086A; Bethyl Laboratories), anti-Rbbp5 pAb (act#A300-109A; Bethyl Laboratories) and anti-Suz12 mAb (cat#3737; Cell Signaling Technology). All antibodies were diluted and used according to the manufacturer’s protocol. CD4 T-cell stimulation and differentiation in vitro Naive CD4 T (CD44 low CD62L high CD25 negative ) cells were prepared using a CD4 + CD62L + T-cell isolation kit II (Miltenyi Biotec). Naive CD4 T cells (1.5 × 10 6 ) were stimulated with immobilized anti-TCR-β mAb (3 μg ml −1 , H57-597, BioLegend) and an anti-CD28 mAb (1 μg ml −1 , 37.5, BioLegend) for 2 days under the conditions indicated. Next, cells were transferred to a new plate and cultured further in the presence of cytokines. Cytokine conditions were as follows: IL-2 (T H ) conditions: IL-2 (2.5 ng ml −1 ); neutral conditions: IL-2 (2.5 ng ml −1 ), anti-IL-4 mAb (5 μg ml −1 , 11B11, BioLegend) and anti-IFN-γ mAb (5 μg ml −1 , R4-6A2, BioLegend). Intracellular staining of cytokines The cells that were differentiated in vitro were stimulated with immobilized anti-TCR-β mAb (3 μg ml −1 , H57-597, BioLegend) for 6 h with monensin (2 μM), and intracellular staining was performed as described. Flow cytometric analysis (FACS) was performed using a FACS Calibur (BD Biosciences), and results were analysed using FlowJo software (Tree Star). ELISA and MILLIPLEX assay The cells were stimulated with immobilized anti-TCR-β mAb for 16 h. The amounts of cytokines and OPN in the supernatants were determined by ELISA, as described. The amounts of chemokines were determined using an MILLIPLEX assay kit according to the manufacturer’s protocol (EMD-Millipore). Quantitative reverse transcriptase polymerase chain reaction Total RNA was isolated using TRIZOL Reagent, and cDNA was synthesized using the Superscript VILO cDNA synthesis kit (Life Technologies). Quantitative RT-PCR was performed as described, using Step One Plus Real-Time PCR Systems (Life Technologies). Primer sequences can be found in the Supplementary Methods . DNA microarray analysis The gene expression profiles of the Menin KO naive CD4 T cells cultured under IL-2-conditions were analysed using the Agilent Whole Mouse 44K Array. The raw data were subjected to log2 transformation and normalized using the Subio Platform (Subio). Pull-down assay Naive CD4 T cells were cultured under T H conditions for 7 days. Then, the cells were pelleted, resuspended in buffer C (20 mM HEPES (pH7.9), 420 mM NaCl, 1.5 mM MgCl 2 , 0.2 mM EDTA, 1 mM dithiothreitol, 0.1% Nonidet P-40, 1 mM Na 2 VO 3 , 1 mM NaF, 1 mM β-glycerophosphate, 1 mM phenylmethylsulfonyl fluoride) and lysed on ice for 15 min. Insoluble material was removed by centrifugation. The supernatant was diluted 1:3 with buffer D (buffer C without NaCl). The lysates were incubated with 10 μg of poly(dI-dC)-poly(dI-dC) (#11-219-847, Roche) and streptavidin-agarose (#16-126, MILLIPRE) carrying indicated biotinylated oligonucleotides for 40 min at 4 °C. The bound proteins were eluted by adding SDS sample buffer and separated on a sodium dodecyl sulphate polyacrylamide gel and then subjected to immunoblotting with specific antibodies. Full size blots can be found in Supplementary Fig. 11 . The NF-κB consensus oligonucleotide probes for the pull-down assay 5′-AGTTGAGGGGACTTTCCCAGGC-3′. Retrovirus-mediated gene transfer Retrovirus infection was performed using pMXs-IRES-hNGFR vector and a Plat-E packaging system, which is kindly, provided by Dr Toshio Kitamura (University of Tokyo, Japan). pMX-Bach2-IRES-hNGFR was constructed by inserting mouse Bach2 cDNA into the multi-cloning site of pMxs-IRES-hNGFR. Virus supernatant was concentrated by centrifugation (8,000 g , 16 h) and added to the T H cell cultures on day 2. After culturing for three more days, the infected cells were detected with anti-human NGFR-PE mAb (ME20.4-1.H4, Miltenyi Biotec). The hNGFR-positive infected cells were purified using an anti-PE microbeads (#130-048-801, Miltenyi Biotec) and an AutoMACS device (Miltenyi Biotec). Analysis of cell viability The WT or Menin KO naïve CD4 T cells were cultured under IL-2-conditions for 7 days and then 10 μM EdU was added for 45 min. EdU incorporation was determined using a Clik-iT EdU Alexa Fluor 488 Flow Cytometry Assay Kit #C35002 (Life Technologies). Cell death was detected using an FITC AnnexinV Apoptosis Detection Kit #556547 (BD Biosciences). SA β-galactosidase assay was performed on day 10 using a Senescence β-Galactosidase Staining Kit #9860 (Cell Signaling Technology). ChIP assay and ChIP-seq The Magna ChIP kit was used according to the manufacturer’s protocol (EMD-Millipore). Samples for ChIP-seq were prepared according to the manufacturer’s protocol (Illumina) and were sequenced using a Genome Analyzer IIx (Illumina). The obtained reads were mapped on the mouse reference genome sequence (9 mm) using the Bowtie 0.12.7 software program. Peak calling was performed using the MACS 1.4.2. software program. To visualize the ChIP sequencing results, the data were converted to a wiggle file format at a 25-base resolution and uploaded to the Subio platform (Subio, Japan). Adoptive transfer For in vivo expansion assay of the antigen-specific CD4 T cells, CD4 T cells from DO11.10 TG mice were sorted using an AutoMACS and transplanted into BALB/c mice. Then the mice were immunized i.p. with 100 μg OVA plus lipoplysaccharide (10 μg). OVA-TCR + cells were detected using the KJ1-26 mAb. To assess the survival of Menin KO T H cells in vivo , the CD45.1 WT or CD45.2 Menin KO naive CD4 T cells were cultured under T H (IL-2) conditions. The WT (CD45.1) and Menin KO (CD45.2) effector CD4 T cells were mixed 1:1 (5 × 10 6 cells each) and transferred into the TCR-βδ KO mice. The ratio of CD45.1 to CD45.2 CD4 T cells was determined using FACS, at 4 weeks after transfer. OVA-induced allergic airway inflammation The WT and Menin KO mice were immunized i.p. with 100 μg OVA in 2 mg of aluminium hydroxide gel (day 0) and challenged with OVA in saline intranasally (100 μg/mouse) on days 8 and 10. Two days later, BAL-fluid cells and lung samples were prepared for histological examination (H&E staining). Infection with Listeria monocytogenes WT and Menin KO mice were infected with Listeria monocytogenes (LM) (EGD strain: 1 × 10 3 CFU) intraperitoneally (primary infection), then reinfected with LM (5 × 10 3 CFU) 14 days after the primary infection (secondary infection). The bacterial burden in the spleen was determined 3 days after each episode of infection. Generation of senescent effector CD4 T cells KJ1 + naive CD4 T cells obtained from DO11.10 OVA-specific TCR TG mice were stimulated with plate bound anti-TCR-β mAb plus anti-CD28 mAb in the presence of IL-2 for 2 days, after which the cells were further expanded with IL-2 for an additional 3 days in vitro . The cells were then transferred intravenously into syngeneic BALB/c nu/nu recipient mice. Four weeks after the transfer, KJ1 + -transferred CD4 T cells were recovered from the spleens of the recipient mice and expanded using the same method as in the primary stimulation and used as a senescent effector CD4 T (sT H ) cell’. Statistical analysis Student’s t -test was used for the statistical analyses. Accession codes: The microarray and ChIP sequencing data were deposited in the NCBI Gene Expression Omnibus (GEO) database under accession numbers GSE49968 and GSE53831 , respectively. How to cite this article: Kuwahara, M. et al. The Menin–Bach2 axis is critical for regulating CD4 T-cell senescence and cytokine homeostasis. Nat. Commun. 5:3555 doi: 10.1038/ncomms4555 (2014).